Targeted genomic rearrangements using CRISPR/Cas technology Genomic rearrangements are frequently observed in cancer cells but have been difficult to generate in a highly specific manner for functional analysis. Here we report the application of CRISPR/Cas technology to successfully generate several types of chromosomal rearrangements implicated as driver events in lung cancer, including the CD74-ROS1 translocation event and the EML4-ALK and KIF5B-RET inversion events. Our results demonstrate that Cas9-induced DNA breaks promote efficient rearrangement between pairs of targeted loci, providing a highly tractable approach for the study of genomic rearrangements. Cancer cells are characterized by abnormalities in chromosome number and structure, such as genomic rearrangements that can result in the inappropriate expression or activation of oncogenes [1] . While many novel cancer-associated rearrangements continue to be identified, it remains difficult to accurately model these events for functional analyses. The ability to efficiently generate specific rearrangements would greatly improve our understanding of how structural variations in the genome arise and how each of these events contributes to disease pathogenesis. The CRISPR (clustered regularly interspaced short palindromic repeats) system has recently been adapted to provide site-specific DNA recognition and cleavage through a customizable RNA guide [2] , [3] , [4] , [5] . Cas9 from Streptococcus pyogenes recognizes a 20 nucleotide target sequence immediately upstream of the requisite protospacer-adjacent motif sequence NGG [6] . Co-expression of the Cas9 enzyme and a chimeric single-guide RNA (sgRNA) results in Cas9-induced double-strand breaks (DSBs) at the targeted genomic sequence [6] ( Fig. 1a ). We hypothesized that the high efficiency of DNA cleavage mediated by Cas9 would facilitate the formation of rearrangements in a targeted manner. 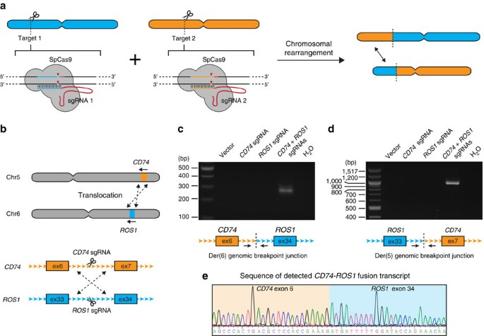Figure 1: Cas9-induced DNA breaks promote interchromosomal translocations. (a) Schematic depicting the overall strategy for generating chromosomal rearrangements. Cas9 fromS. pyogenes(SpCas9) is co-expressed with two single-guide RNAs (sgRNA 1 and 2) that direct DNA cleavage at each targeted genomic site. (b) TheCD74-ROS1rearrangement results from a translocation between chromosomes 5 and 6. Shown are the intronic sites where Cas9 was targeted. (c,d) PCR detection of the (c)CD74-ROS1Der(6) and (d)ROS1-CD74Der(5) genomic breakpoint junctions from HEK 293T cells in which Cas9 was expressed with no sgRNA (vector),CD74sgRNA alone,ROS1sgRNA alone, or bothCD74andROS1sgRNAs. (e) Sequence chromatogram of the detectedCD74-ROS1fusion transcript from cells in which Cas9 and bothCD74andROS1sgRNAs were expressed. Data shown are representative results from a total of three independent experiments. Figure 1: Cas9-induced DNA breaks promote interchromosomal translocations. ( a ) Schematic depicting the overall strategy for generating chromosomal rearrangements. Cas9 from S. pyogenes (SpCas9) is co-expressed with two single-guide RNAs (sgRNA 1 and 2) that direct DNA cleavage at each targeted genomic site. ( b ) The CD74-ROS1 rearrangement results from a translocation between chromosomes 5 and 6. Shown are the intronic sites where Cas9 was targeted. ( c , d ) PCR detection of the ( c ) CD74-ROS1 Der(6) and ( d ) ROS1-CD74 Der(5) genomic breakpoint junctions from HEK 293T cells in which Cas9 was expressed with no sgRNA (vector), CD74 sgRNA alone, ROS1 sgRNA alone, or both CD74 and ROS1 sgRNAs. ( e ) Sequence chromatogram of the detected CD74-ROS1 fusion transcript from cells in which Cas9 and both CD74 and ROS1 sgRNAs were expressed. Data shown are representative results from a total of three independent experiments. Full size image Here we specifically investigate whether pairs of DSBs induced by RNA-guided Cas9 would be sufficient to generate chromosomal translocations and inversions ( Fig. 1a ). We model several genomic rearrangements known as driver events in lung adenocarcinoma and representing a variety of rearrangement types. We find that DNA cleavage by Cas9 at two genomic loci results in detectable levels of rearrangement between the targeted regions. DNA rearrangement also results in expression of the expected fusion transcripts and protein products, demonstrating that CRISPR/Cas technology is a highly practical tool for the study of genomic rearrangements. In lung adenocarcinoma, ROS1 is involved in translocations that result in in-frame fusions with CD74 or SLC34A2 (refs 7 , 8 , 9 ). We first attempted to generate the CD74-ROS1 rearrangement, which arises through a translocation between CD74 on chromosome 5 and ROS1 on chromosome 6 ( Fig. 1b ). We designed sgRNAs targeting intron 6 of CD74 and intron 33 of ROS1 ( Fig. 1b ), which were then co-expressed with Cas9 in HEK 293T cells. Cleavage of each targeted region was highly efficient, as assessed by the formation of indels using the Surveyor assay ( Supplementary Fig. 1a ). Using primers spanning the expected breakpoint junction, we detected translocations occurring in cells expressing both CD74 and ROS1 sgRNAs, but not in cells expressing only a single targeting sgRNA ( Fig. 1c,d ; Supplementary Fig. 5a,b ). Sequencing of breakpoints confirmed formation of the CD74-ROS1 translocation event and we observed junction types resulting from both precise joining of predicted cleavage sites and those containing short deletions that likely result from nucleolytic processing of DNA ends during DSB repair ( Supplementary Fig. 2a,b ). In addition, we detected expression of the predicted CD74-ROS1 fusion transcript from complementary DNA samples using primers spanning the junction between CD74 exon 6 and ROS1 exon 33 ( Fig. 1e ; Supplementary Fig. 2c ). We were also able to generate the same CD74-ROS1 translocation in non-transformed immortalized lung epithelial cells (AALE) [10] , which represent a more relevant cellular context for studying the CD74-ROS1 rearrangement event ( Supplementary Fig. 3, 5c,d ). Collectively, these results demonstrate that Cas9-induced DSBs are sufficient to promote translocations between targeted chromosomes in multiple cell types. Next, we sought to determine whether Cas9-mediated DNA cleavage could promote the formation of intrachromosomal inversions. We chose to model the EML4-ALK and KIF5B-RET rearrangements observed in lung cancer, which represent two different types of inversion events. EML4-ALK is the result of a paracentric inversion of chromosome 2p (ref. 11 ), while KIF5B-RET is the result of a pericentric inversion across the two arms of chromosome 10 (refs 9 , 12 , 13 , 14 ) ( Fig. 2a,f ). We first selected target sites that were in the immediate vicinity of intronic breakpoints identified in patient samples containing the EML4-ALK [11] and KIF5B-RET [13] rearrangements. Introduction of constructs expressing Cas9 and each targeting sgRNA into HEK 293T cells resulted in efficient site-specific cleavage, as detected by indel formation ( Supplementary Fig. 1b,c ). For both EML4-ALK and KIF5B-RET , the expected inversions were only detected in cells expressing Cas9 along with the appropriate pair of sgRNAs, as compared with control cells expressing only one sgRNA ( Fig. 2b,g ; Supplementary Fig. 5e,g ). EML4-ALK and KIF5B-RET fusion transcripts were also detected only when both sites were targeted ( Fig. 2c,h ; Supplementary Fig. 5f,h ), and matched the predicted sequence ( Fig. 2d,i ; Supplementary Fig. 4 ). In addition, among single-cell clones that were derived from cells transfected with the combination of EML4 and ALK sgRNAs, we identified several positive clones that expressed the EML4-ALK fusion protein ( Fig. 2e ). 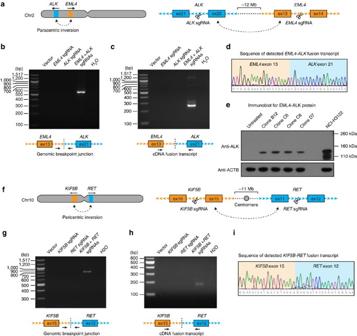Figure 2: Cas9 can be targeted to generate paracentric and pericentric intrachromosomal inversions. (a) TheEML4-ALKrearrangement results from a paracentric inversion in chromosome 2. Shown are the intronic sites where Cas9 was targeted. (b,c) PCR detection of theEML4-ALK(b) genomic breakpoint junction and (c) fusion transcript from HEK 293T cells in which Cas9 was expressed with no sgRNA (vector),EML4sgRNA alone,ALKsgRNA alone, or bothEML4andALKsgRNAs. (d) Sequence chromatogram of the detectedEML4-ALKfusion transcript from cells in which Cas9 and bothEML4andALKsgRNAs were expressed. (e) Western blot for EML4-ALK protein expression in single clones of 293T cells that were untreated, or in which Cas9 and bothEML4andALKsgRNAs were expressed. NCI-H3122 cells are shown as a positive control. (f) TheKIF5B-RETrearrangement results from a pericentric inversion in chromosome 10. Shown are the intronic sites where Cas9 was targeted. (g,h) PCR detection of theKIF5B-RET(g) genomic breakpoint junction and (h) fusion transcript from HEK 293T cells in which Cas9 was expressed with no sgRNA (vector),KIF5BsgRNA alone,RETsgRNA alone, or bothKIF5BandRETsgRNAs. (i) Sequence chromatogram of the detectedKIF5B-RETfusion transcript from cells in which Cas9 and bothKIF5BandRETsgRNAs were expressed. Data shown are representative results from a total of three independent experiments. Figure 2: Cas9 can be targeted to generate paracentric and pericentric intrachromosomal inversions. ( a ) The EML4-ALK rearrangement results from a paracentric inversion in chromosome 2. Shown are the intronic sites where Cas9 was targeted. ( b , c ) PCR detection of the EML4-ALK ( b ) genomic breakpoint junction and ( c ) fusion transcript from HEK 293T cells in which Cas9 was expressed with no sgRNA (vector), EML4 sgRNA alone, ALK sgRNA alone, or both EML4 and ALK sgRNAs. ( d ) Sequence chromatogram of the detected EML4-ALK fusion transcript from cells in which Cas9 and both EML4 and ALK sgRNAs were expressed. ( e ) Western blot for EML4-ALK protein expression in single clones of 293T cells that were untreated, or in which Cas9 and both EML4 and ALK sgRNAs were expressed. NCI-H3122 cells are shown as a positive control. ( f ) The KIF5B-RET rearrangement results from a pericentric inversion in chromosome 10. Shown are the intronic sites where Cas9 was targeted. ( g , h ) PCR detection of the KIF5B-RET ( g ) genomic breakpoint junction and ( h ) fusion transcript from HEK 293T cells in which Cas9 was expressed with no sgRNA (vector), KIF5B sgRNA alone, RET sgRNA alone, or both KIF5B and RET sgRNAs. ( i ) Sequence chromatogram of the detected KIF5B-RET fusion transcript from cells in which Cas9 and both KIF5B and RET sgRNAs were expressed. Data shown are representative results from a total of three independent experiments. Full size image To estimate the efficiency of the induced EML4-ALK and KIF5B-RET rearrangements, we developed a flow cytometric assay to quantify ALK or RET protein expression at the single-cell level. Untreated HEK 293T cells do not express appreciable amounts of either ALK or RET, allowing the levels of these proteins to serve as surrogate markers of successful rearrangement. For the EML4-ALK rearrangement, we observed increased ALK expression in ~8% of cells treated with both EML4 and ALK sgRNAs, compared with 1% or less of cells treated with single sgRNAs or no sgRNAs ( Fig. 3a ), while for the KIF5B-RET rearrangement, we observed increased RET expression in ~1.6% of cells treated with both KIF5B and RET sgRNAs, compared with less than 0.5% of cells treated with single sgRNAs or no sgRNAs ( Fig. 3b ). Taken together, our results demonstrate that intrachromosomal inversions involving a single arm or occurring across both arms can be readily generated using the CRISPR/Cas system. 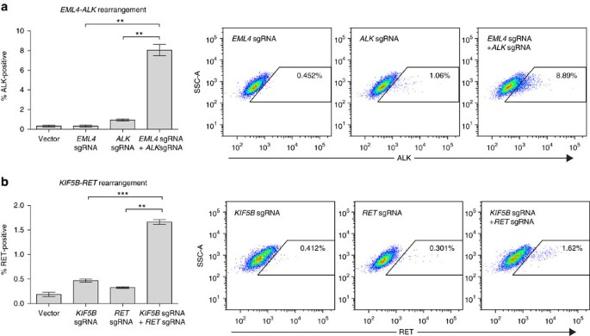Figure 3: Estimated efficiencies of inducingEML4-ALKandKIF5B-RETrearrangements. HEK 293T cells transfected with Cas9 and no sgRNA (vector), a single sgRNA, or a pair of sgRNAs were stained for either (a) ALK or (b) RET protein to estimate the percentage of cells with inducedEML4-ALKorKIF5B-RETrearrangements, respectively. All values represent means of at least three independent experiments ±s.e.m. Means were compared by pairedt-test (**P<0.01, ***P<0.001). Also shown are dotplots from a representative experiment for each rearrangement. Figure 3: Estimated efficiencies of inducing EML4-ALK and KIF5B-RET rearrangements. HEK 293T cells transfected with Cas9 and no sgRNA (vector), a single sgRNA, or a pair of sgRNAs were stained for either ( a ) ALK or ( b ) RET protein to estimate the percentage of cells with induced EML4-ALK or KIF5B-RET rearrangements, respectively. All values represent means of at least three independent experiments ±s.e.m. Means were compared by paired t -test (** P <0.01, *** P <0.001). Also shown are dotplots from a representative experiment for each rearrangement. Full size image We have found that targeted DNA DSBs induced by Cas9 can promote genomic rearrangements of several types, including interchromosomal translocations and intrachromosomal inversions. Previously, it has been reported that chromosomal rearrangements can also be generated using meganucleases, zinc-finger nucleases and transcription activator-like effector nucleases [15] , [16] , [17] . While all of these tools have revolutionized our ability to manipulate the genome, the CRISPR/Cas9 system offers several unique advantages. The ease with which sgRNAs can be designed and cloned makes the CRISPR system well suited for high-throughput screening experiments. Also, the ability to multiplex Cas9 targeting opens up the possibility of studying more complex combinations of rearrangements observed in cancer genomes, such as those resulting from chromothripsis [18] or chromoplexy [19] . In addition, while off-target recognition and cleavage by Cas9 may result in non-specific chromosomal rearrangements, these unintended effects could be minimized by generating DSBs using a ‘double-nicking’ strategy [20] , [21] or targeting with shorter 17nt sgRNAs that exhibit greater specificity [22] . The rearrangements and inversions induced in this study are most likely occurring through the non-homologous end-joining (NHEJ) pathway of DSB repair, as they involve the joining of mismatched ends. We did not detect regions of significant homology between the targeted DNA regions, suggesting that alternative forms of repair, such as non-allelic homologous recombination, are unlikely to be responsible for generating the induced rearrangements. From our analysis of the rearranged genomic breakpoint junctions, we observed a high frequency of exact fusion events, which may be explained by the mechanism of Cas9-mediated DNA cleavage. It has been described previously that Cas9 generates blunt ends precisely 3 bp upstream of the protospacer-adjacent motif sequence [6] . Since the resulting blunt DNA ends would not require further end-processing before ligation in the NHEJ pathway of repair, rearrangements between Cas9-generated ends may frequently occur as exact fusion events. Similarly, NHEJ-mediated repair of blunt-ended signal joints generated during V(D)J recombination also results in precise error-free fusions [23] . However, the nature of an induced fusion site is also likely to depend on a variety of other factors, such as features specific to the genomic regions that are targeted, the unique properties of the cell lines that are used and the levels of Cas9/sgRNAs that are expressed. We propose that Cas9-mediated targeting of endogenous loci provides a highly useful approach for the study of novel chromosomal rearrangements and their functional significance in human disease. Accurate modelling of rearrangements will provide opportunities to not only study the phenotypic consequences of specific events but also investigate the mechanisms that contribute to structural changes to the genome. CRISPR sgRNA target selection and cloning Suitable sgRNA target sites were manually identified based on the following criteria: an initiating G on the 5′-end, the presence of an NGG motif on the 3′-end, proximity to breakpoints previously reported in patient samples (when such information was available) and sequence uniqueness by BLAST search. Oligos encoding the targeting sequence were then annealed and ligated into the BbsI sites of pX330 (ref. 3 ; Addgene #42230). Sequences of sgRNA oligos are listed in Supplementary Table 1 . Cell transfection and DNA extraction HEK 293T cells were plated the day before transfection at 10 6 cells per well of a six-well plate. On the day of transfection, the medium was replaced to antibiotic-free DMEM/10% fetal bovine serum. Cells were treated with 25 μM of chloroquine and transfected with a total of 2 μg of DNA by the calcium phosphate method (CalPhos Kit, Clontech #631312). Transfection efficiencies were estimated by transfection of a green fluorescent protein reporter plasmid in each experiment and averaged 85–95%. For transfection of AALE cells, 5 × 10 5 cells were nucleofected with a total of 2 μg of DNA using the Basic Epithelial Cell Nucleofector Kit (Lonza VPI-1005) and the T13 setting. Media was replaced the following day and cells were harvested ~72 h post transfection. DNA was extracted from cells using Quickextract DNA extraction solution (Epicentre #QE09050) and diluted to 10 ng μl −1 for subsequent PCR analyses. RNA extraction and reverse transcription–PCR Total RNA was purified from cells using the NucleoSpin RNA kit (Machery-Nagel #740955). First-strand cDNA synthesis was subsequently carried out on 1 μg of total RNA with the iScript cDNA Synthesis Kit (Bio-Rad #170-8891). PCR-based detection of genomic breakpoints and cDNA fusions PCR amplification was carried out using Q5 high-fidelity DNA polymerase (NEB #M0491). PCR products were electrophoresed on 2% TBE gels and purified using the Nucleospin Gel and PCR Clean-up kit (Machery-Nagel #740609). Purified PCR products were directly sequenced using the forward PCR primer. CD74-ROS1 and ROS1-CD74 genomic breakpoint PCR products were cloned into pJET1.2 using the CloneJET PCR Cloning Kit (Thermo Scientific #K1231) and individual clones were sequenced. PCR primers are listed in Supplementary Table 1 . Isolation of EML4-ALK clones and western blotting HEK 293T cells transfected with both EML4 and ALK sgRNAs were single cell cloned by limiting dilution in 96-well plates. Individual clones were screened by PCR for the EML4-ALK genomic rearrangement. PCR-positive clones were subsequently screened by western blotting for ALK expression using standard procedures. Cells were lysed in RIPA buffer and lysates were separated on 4–12% Bis-Tris NuPage gels (Invitrogen). After transferring to polyvinylidene fluoride membranes, blots were probed with antibodies against ALK (Cell Signaling Technology #3633, 1:1,000) or ACTB (Cell Signaling Technology #8457, 1:1,000). Surveyor nuclease assay Genomic regions surrounding sgRNA-targeted sites were amplified by PCR (see Supplementary Table 1 for primer sequences). PCR products were gel extracted or purified directly using the Nucleospin Gel and PCR Clean-Up Kit (Machery-Nagel, #740609). Approximately 200–400 ng of each PCR product was then denatured and re-annealed in 20 μl total volume containing Pfu Turbo reaction buffer, as specified in the Surveyor Mutation Detection Kit protocol (Transgenomics #706020). Next, 2 μl of 0.15 M MgCl 2 , 1 μl of Surveyor enhancer solution, and 1 μl of Surveyor nuclease was added and the mixture was incubated at 42 °C for 60 min. Reactions were stopped with addition of 2 μl of Stop solution and separated on 2% TBE agarose gels. Intracellular staining for ALK and RET Cells were washed in PBS and fixed with 2% paraformaldehyde in PBS for 10 min. at 37 °C. After washing in PBS, cells were permeabilized in cold 90% methanol for 30 min on ice. Cells were then washed in 0.5% BSA in PBS and stained with anti-ALK (Cell Signaling Technology, #3633P, 1:400) or anti-RET (Cell Signaling Technology, #3223S, 1:50) for 1 h at room temperature, followed by a wash in 0.5% BSA in PBS, and staining with anti-rabbit Alexa Fluor 488 secondary antibody (Life Technologies, #A11070, 1:500) for 30 min at room temperature. After a final wash, cells were resuspended in PBS and analysed on a BD LSR Fortessa flow cytometer. How to cite this article: Choi, P. S. and Meyerson, M. Targeted genomic rearrangements using CRISPR/Cas technology. Nat. Commun. 5:3728 doi: 10.1038/ncomms4728 (2014).